Electron-beam-assisted superplastic shaping of nanoscale amorphous silica As structural and functional members, glassy oxides are widely used in today's electronic and optical devices, and microelectromechanical or nanoelectromechanical systems, fabricated in the forms of thin films, fibers, wires, pillars, particles and cantilever beams [1] , [2] . Owing to the difficulties in their synthesis and assembly, the as-prepared objects may not have the desired shape. Therefore, one may want to plastically deform them locally to alter their dimensions and configuration. However, such glasses are characterized by covalent and ionic bonding, and hence brittle materials. The silicon dioxide glass (and amorphous silica) is typical of such materials [3] , [4] that do not exhibit ductility at room temperature (RT) to allow plastic deformation after their fabrication into structures/devices. This is because the silica glass has a glass-transition temperature T g as high as 1,373 K [5] , [6] , and RT is just too low a temperature for viscous flow to contribute significantly to the accommodation of the imposed deformation rate. Any mechanical re-shaping is thus practically impossible near RT. Hot deformation/shaping is not a viable option either, because the substantial heating would undoubtedly damage the surrounding components. New opportunities arise, when the brittle objects in question are on nanoscale and energetic beams such as the e-beam in a conventional electron microscope can be used to irradiate through them. Previously, e-beam has been exploited for the irradiation-assisted engineering of nanoscale materials [7] , mostly by making use of intense beams focused onto a spot (enormous beam current densities can be achieved, up to 300 A cm −2 with beams from thermal electron guns and 10 5 A cm −2 from field emission guns (FEGs)). Such highly localized beams can be used to tailor nanomaterials for the patterning of ultrathin films [8] , the fabrication of nanodots [9] , the self-organization of ensembles of nanoclusters [10] , the transformation of spherical nanocolloids into other shapes, the creation of metallic nanoparticles in dielectric matrices, the altering of the properties of nanotubes [7] and the drilling, cutting and welding of nano-objects [11] . However, processing with low beam intensities without obvious rise in sample temperature, for the purpose of facilitating plastic deformation under applied stresses, has not yet been explored, let alone quantitatively studied. Under high stresses, a glass can plastically deform through the bond breaking and bond-switching processes that mediate the rotation and migration of atomic clusters [12] , [13] . With e-beam illumination, oxygen vacancies and ionization damage, including dangling bonds, are constantly induced throughout the material, owing to the interaction of the atoms with the incoming high-energy electrons. This is expected to significantly enhance the flow mechanism (see Discussion ). In other words, the e-beam introduces additional 'flow defects' to facilitate large plastic deformation that is not possible in bulk samples. In fact, superplastic flow can be achieved near RT; here, we show this e-beam-assisted superplastic shaping of amorphous silica using in situ experiments inside a transmission electron microscope (TEM). In situ compression tests The as-fabricated amorphous silica, even when on 100 nm scale, is known to be unable to sustain large plastic flow [14] , [15] . Our in situ tests reveal a surprisingly different behavior, with the help from high-energy electrons. Figures 1 , 2 , 3 show the typical deformation response of amorphous silica nanoparticles in compression tests inside a JEOL 2100F TEM. Six particles have been tested, yielding reproducible results. 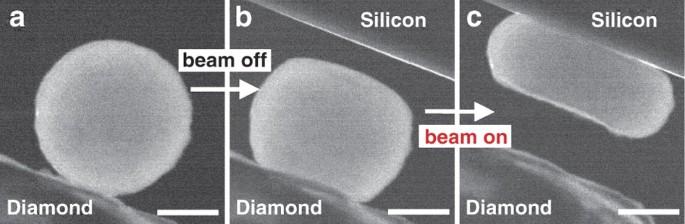Figure 1: Nanocompression of amorphous silica particle inside a transmission electron microscope (TEM). Two consecutive compression runs were performed with the electron beam being off and on, respectively. Panelsa–cshow the centered dark-field images. Ina, the particle is adhered to the diamond punch and the silicon has not moved into the picture. Inb, the particle is imaged after it has been pressed with the beam off. Subsequently, with the beam on, the particle can be compressed into a pancake with a moderate force, as seen inc. The scale bars are for 200 nm. Figure 1a displays the centered dark-field image of a silica particle with a diameter of 510 nm before the compression test. After imaging for the positioning of the sample and the diamond flat punch, the beam was blocked off with the condenser lens aperture, and the silica particle was compressed with the Hysitron PicoIndenter [16] , [17] (see Methods ). The particle is plastically deformable ( Fig. 1b ) apparently because of the e-beam irradiation it had experienced during the imaging. Three load-partial unload cycles were performed under this beam-off condition; see the load-displacement traces in Fig. 2 . After ∼ 40 percent compression [16] (defined as the compression displacement of the particle, Z , divided by its diameter, D ), the beam was brought on the sample to image the particle ( Fig. 1b ), which reveals no fracture and crystallization during the deformation. By assuming a circular cross-sectional contact area, the contact pressure at this point (peak force 790 μN divided by the punch–particle contact area at the measured contact diameter of 330 nm) is estimated to be 9.2 GPa. This high stress has reached the ultimate strength of silica glass at such a size (10 GPa for a nanowire (NW) diameter of 300 nm [14] ), and further deformation becomes difficult as the contact area keeps increasing and the force is already approaching the capacity limit of the Hysitron Picoindenter. On unloading at point b in Fig. 2 , the total plastic (not recoverable as in elastic deformation or reversible phase transformation [18] ) percent compression was 27%. Surprisingly, the plastic flow of the glass was continuous and smooth, with no sign of shear banding or cracking. Figure 1: Nanocompression of amorphous silica particle inside a transmission electron microscope (TEM). Two consecutive compression runs were performed with the electron beam being off and on, respectively. Panels a – c show the centered dark-field images. In a , the particle is adhered to the diamond punch and the silicon has not moved into the picture. In b , the particle is imaged after it has been pressed with the beam off. Subsequently, with the beam on, the particle can be compressed into a pancake with a moderate force, as seen in c . The scale bars are for 200 nm. 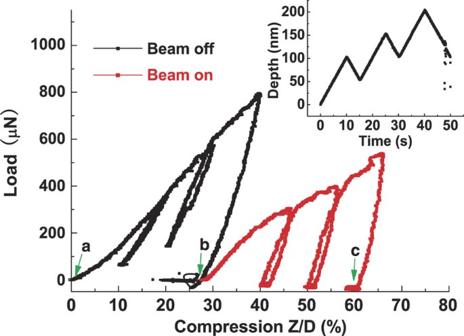Figure 2: Load versus percent compression for the nanocompression test of amorphous silica nanoparticle. The points (a, b and c) correspond to the three panels inFig. 1. The percent compression is defined as the depth traveled by the diamond punch divided by the diameter of the particle,D,∼510 nm. The inset shows the programmed loading–partial unloading procedure, which is in displacement-controlled mode with a rate of 10 nm s−1. The episodes showing decrease in the displacement depthZcorrespond to the unloading segments. The force decreases dramatically with beam on, indicating that the particle becomes much softer under the beam. The force below zero was because of the adherence of the sample to the diamond punch and silicon substrate after compression. Full size image Figure 2: Load versus percent compression for the nanocompression test of amorphous silica nanoparticle. The points (a, b and c) correspond to the three panels in Fig. 1 . The percent compression is defined as the depth traveled by the diamond punch divided by the diameter of the particle, D , ∼ 510 nm. The inset shows the programmed loading–partial unloading procedure, which is in displacement-controlled mode with a rate of 10 nm s −1 . The episodes showing decrease in the displacement depth Z correspond to the unloading segments. The force decreases dramatically with beam on, indicating that the particle becomes much softer under the beam. The force below zero was because of the adherence of the sample to the diamond punch and silicon substrate after compression. 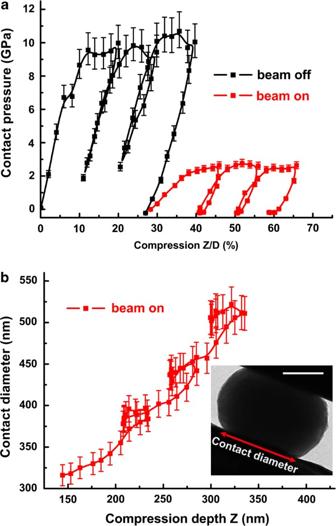Figure 3: Contact pressure (stress) versus percent compression of the amorphous silica particle. Ina, the contact pressure was monitored throughout the beam-off (black) and beam-on (red) compression tests. The videotape records the evolution of the contact diameter throughout the compression; seebfor the beam-on test (the error bar for the contact diameter measurement is ±4%). Assuming circular cross-section, the contact pressure (stress) was then estimated from the contact diameter measured (see the inset inb; the scale bar is 200 nm). For example, at the eventual peak force (530 μN) and 65% compression, the measured contact diameter is 495 nm, as seen inFigure 1c, such that the contact pressure is 2.5 GPa. Full size image Figure 3: Contact pressure (stress) versus percent compression of the amorphous silica particle. In a , the contact pressure was monitored throughout the beam-off (black) and beam-on (red) compression tests. The videotape records the evolution of the contact diameter throughout the compression; see b for the beam-on test (the error bar for the contact diameter measurement is ±4%). Assuming circular cross-section, the contact pressure (stress) was then estimated from the contact diameter measured (see the inset in b ; the scale bar is 200 nm). For example, at the eventual peak force (530 μN) and 65% compression, the measured contact diameter is 495 nm, as seen in Figure 1c , such that the contact pressure is 2.5 GPa. Full size image Much easier flow was observed, with the ensuing beam-on deformation in a second set of in situ experiments ( Fig. 1c ). This set is comprised of another three loading–partial unloading cycles, and the load-percent compression curves (red) are included in Figure 2 . Although the contact area kept increasing, the forces required to deform was at levels considerably lower than those in the beam-off condition. The stress (contact pressure) required to keep the plastic flow going is monitored and found to remain at a steady level of ∼ 2.5 GPa throughout the three cycles (see Fig. 3 and its caption). In the end (corresponding to Fig. 1c and point c in Fig. 2 ), the spherical particle has been shaped into a pancake, with no sign of crystallization, strain localization or cracking. This remarkable deformability is videotaped and shown in Supplementary Movie 1 . Note that the 2.5 GPa stress level is higher than the compressive strength (0.7–1.4 GPa [14] , [19] , [20] ) of bulk silica glass at RT. A key point is that this plastic flow is not achieved because of high sample temperature, as will be discussed in detail in a later sub-section. In situ tensile tests The deformation of the amorphous silica is in fact superplastic. As superplasticity is defined as large uniform elongation in tension, we show this by an in situ tensile experiment, by pulling a single NW inside the TEM. The NW was bridge tangled between two broken parts of the supporting holy carbon film. Under e-beam, a pulling force was generated when the carbon is being illuminated (see Methods ), [21] , [22] and the low-strain-rate ( ∼ 10 −4 per second) tensile deformation was captured in real time. 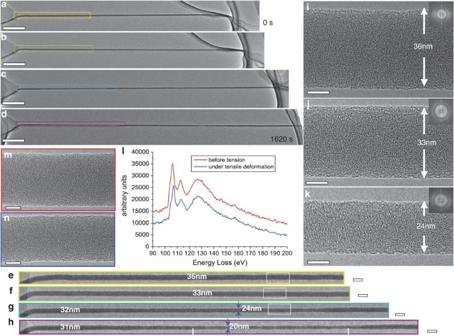Figure 4:In situtransmission electron microscope (TEM) images showing the superplastic tensile elongation of a silica nanowire (NW) under moderate e-beam illumination. Panelsa–dshow the large strains, with magnified images (e–h) corresponding to the color-framed regions. High-resolution electron microscope (HREM) images (i–k) are given for the white-boxed regions, showing uniform and dramatically reduced wire diameter. The insets in (i–k) are selected area diffraction patterns for these regions, confirming the amorphous nature of the material. The red and blue curves inlare the EELS (electron energy loss spectroscopy) spectra taken from the regions inn(before deformation) andm(after 20% elongation), respectively. The dimensions of the scale bars are: (a–d), 500 nm; (e–h), 50 nm; (i–k,m,n), 10 nm. Figure 4a–d show the rather uniform plastic flow experienced by the NW, and Fig. 4e–h are the magnified images corresponding to the respective color-framed regions in Fig. 4a–d . The initial NW diameter was 36 nm before tensile deformation, and decreased to an average of 20.3±0.6 nm in Fig. 4h . At that point, the deformation spreads quite uniformly in the region marked by the two white bars in Fig. 4h . In this particular region ( ∼ 700 nm), the reduction in the cross-sectional area is ∼ 68% on average and approximately uniform; see Fig. 5 for a point-to-point evaluation along the wire length. Assuming constant NW volume, the superplastic elongation is as large as 215%. Figure 4: In situ transmission electron microscope (TEM) images showing the superplastic tensile elongation of a silica nanowire (NW) under moderate e-beam illumination. Panels a – d show the large strains, with magnified images ( e – h ) corresponding to the color-framed regions. High-resolution electron microscope (HREM) images ( i – k ) are given for the white-boxed regions, showing uniform and dramatically reduced wire diameter. The insets in ( i – k ) are selected area diffraction patterns for these regions, confirming the amorphous nature of the material. The red and blue curves in l are the EELS (electron energy loss spectroscopy) spectra taken from the regions in n (before deformation) and m (after 20% elongation), respectively. The dimensions of the scale bars are: ( a – d ), 500 nm; ( e – h ), 50 nm; ( i – k , m , n ), 10 nm. 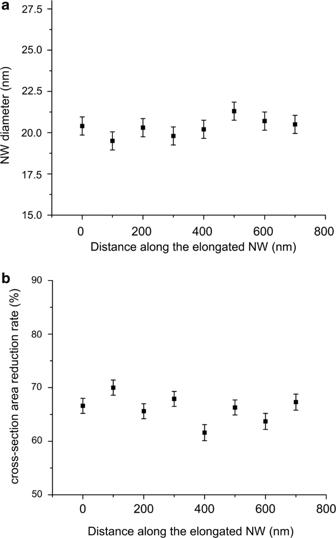Figure 5: Approximately uniform nanowire diameter and cross-sectional area during the superplastic elongation. The silica nanowire (NW) before and after tensile elongation can be found inFig. 4e and h, respectively. Panelapresents the NW diameters measured every 100 nm along the wire inFig. 4h(between the two white bars, left bar at 0 nm and right bar at 700 nm). The average diameter of the elongated NW is calculated to be 20.3 nm, with a standard deviation of 0.55 nm (used for the error bar ina). The corresponding cross-section area reduction (relative to the original area) is plotted inb, with an average value of 68.2%. Assuming that the NW volume remains the same during the deformation, the calculated elongation in this gauge length is 215%. Full size image Figure 5: Approximately uniform nanowire diameter and cross-sectional area during the superplastic elongation. The silica nanowire (NW) before and after tensile elongation can be found in Fig. 4e and h , respectively. Panel a presents the NW diameters measured every 100 nm along the wire in Fig. 4h (between the two white bars, left bar at 0 nm and right bar at 700 nm). The average diameter of the elongated NW is calculated to be 20.3 nm, with a standard deviation of 0.55 nm (used for the error bar in a ). The corresponding cross-section area reduction (relative to the original area) is plotted in b , with an average value of 68.2%. Assuming that the NW volume remains the same during the deformation, the calculated elongation in this gauge length is 215%. Full size image The high-resolution electron microscope (HREM) images ( Fig. 4i–k ), corresponding to the white-framed regions in Fig. 4e–g , clearly show the rather smooth surfaces, the absence of severe localization of strain, as well as the amorphous nature of the NW without deformation/beam-induced crystallization. The amorphous structure of the deformed silica NW is also confirmed by the corresponding selected area diffraction patterns displayed in the insets of Fig. 4i–k . Electron energy loss spectroscopy (EELS) analysis was also conducted: the two Si-L 2,3 edge EELS spectra in Fig. 4l were taken before deformation ( Fig. 4m ) and after 20% deformation ( Fig. 4n ). Both spectra show the Si-L 2,3 ionization edge starting at about 106 eV, indicating typical amorphous silica. Apparently, the large tensile ductility did not derive from a crystallization process or a large composition excursion. We first discuss the key issue of deformation temperature under the e-beam. Significant beam heating is not expected in the sample, for many reasons. First, the e-beam current intensity (≤1.8×10 −2 A cm −2 ) we used for both the in situ compressive and tensile deformation, and even that (4 A cm −2 ) for high-resolution imaging of the NW shown in Figure 4 , is rather low, several orders of magnitude lower than those used previously for beam-induced creation of holes, cutting, welding and evaporation [11] , or for beam-induced nanoscale viscous flow of silica [23] , [24] , [25] . Second, we also have good thermal contact. This was achieved for the NW as it tangles with the carbon-supporting film (the contact was able to sustain very large tensile forces), as well as for the nanoparticle through repeated (load–unload–reload) high-pressure pressing that smoothed out asperities and adhered the diamond punch to the sample, during (and in fact even before) the beam-on tests. Indeed, there is a large and intimate contact (diameter ∼ 330 nm, after the beam-off tests; see Fig. 1 , 2 , 3 , Supplementary Movie 1 ) of the sample with the compressing diamond punch and silicon substrate, under high pressure (2.5 GPa). Third, to quantitatively estimate the temperature rise inside the sample due to e-beam irradiation, we have carried out a thermal conduction analysis, which is presented here. The origin of the temperature rise is the energy loss of the 200 keV electrons when they travel through the material. The average energy loss (per unit length) of an electron in the material is Q = Q c +Q r , where Q c is the collision stopping power (0.51 eV nm −1 in this case [26] ), and Q r is the radiative stopping power (1.57×10 −3 eV nm −1 [26] ) due to bremsstrahlung. The e-beam energy is transferred to the sample at an energy density rate of H=QJ/e =9×10 10 W m −3 , where J is the electron current density (1.8×10 −2 A cm −2 ) and e is the elementary charge (1.6×10 −19 C ). If the sample was completely isolated, the temperature would increase rapidly with the irradiation time ( t ) following Ht/ρC , where C =703 J kg −1 K −1 is the specific heat of silica and ρ =2.2×10 3 kg m −3 is the mass density. However, the sample is in intimate contact with good heat conductors that are far larger in volume than the sample. The thermal conductivity k , is as large as 3,320 W m −1 K −1 for diamond and 149 W m −1 K −1 for silicon, both much larger than that of silica glass, 1.4 W m −1 K −1 . Because of this and the low J used, the large diamond probe and silicon substrate should have experienced little temperature increase. As a result, the heat accumulated in the sample will be dissipated through the contact interfaces with the diamond and silicon, and when this heat accumulation–dissipation process reaches equilibrium, we have where V is the volume of the sample, G is the contact thermal conductance, A is the total area of the contact interface, which can be calculated from its diameter, and Δ T is the temperature difference at the interface between the sample and the silicon/diamond. G may take a wide range of values depending on the details of the interface. For example, for a solid–solid interface created by vapor deposition or epitaxy, the contact is almost ideal and the conductance can be as high as 10 ∼ 1,000 MW m −2 K −1 ( [27] ). However, for macroscopic rough surfaces, the micron-scale asperity may significantly reduce the “effective contact” that is truly in touch, thus the measured conductance could be very low (for example, <0.01 MW m −2 K −1 ; refs 28 , 29 ). The exact values in the latter case also depend sensitively on the applied pressure as well as the transmitting medium caged in-between the rough surfaces. The G in our case is between the two extremes, but it is expected to be closer to the upper bound. This is because our interface is already at nanometer scale, and any small-scale asperity, when under high pressure, is going to be eliminated because of plastic fit. In fact, the load-displacement curve shows that considerable force is needed to pull the sample and the probe apart after compression, overcoming the adhesion. Also, Fig. 3b and Supplementary Movie 1 demonstrate clearly that the contact is intimate over a rather large area. Contact thermal conductance in several closely related cases have been quantitatively measured before, including the nanoscale contact between a Pt-Rh probe of scanning thermal microscope and various sample surfaces [30] , adhered microcantilevers on the substrate [31] , as well as the contact between wafer-like Al/Si solid surfaces under ∼ 10MPa pressure [32] . They all give contact thermal conductance at least of the order of 1 MW m −2 K −1 . We thus take G= 1 MW m −2 K −1 for the following estimation. Using the measured A and V≈ 7×10 −20 m 3 , equation (1) gives a Δ T as small as 0.1 K. Therefore, the temperature of the sample at the interface is almost pinned at RT. We then consider the temperature around the center of the sample, which could be higher than the interface temperature because of the low thermal conductivity of amorphous silica. At equilibrium, the temperature field inside the sample satisfies Substituting the H value solved above for our e-beam and the k value for silica glass into equation (2), we have Assuming there is a hottest point in the sample interior (e.g., center of the particle or middle of the NW), where the temperature gradient is zero, and the heat flow is outbound towards the contact interfaces, we may use the and the sample dimension to estimate the temperature difference in the sample. The latter is found, because of the very small H and sample size, to be only 10 −3 – ∼ 10 −2 K. In other words, the entire sample remains cold—as cold as the diamond/silicon. The temperature equilibrium established with the surroundings is also evidenced by the little change in the level of the compressing stress (which would otherwise decrease if the particle were isolated and became hotter and hotter, or increase if one assumes that the thermal contact area increases on increasing compression). The small temperature rise in our case is primarily due to the large (relative to the small sample size) and intimate contact area under the compressing diamond/silicon and the very low electron current density. However, if the heat dissipation is limited by isolating the nanoparticle (for example, reducing the contact area), or a much higher current density is used, the temperature rise could be more significant, as shown in previous experiments [33] . In fact, the contact area/volume ratio ( A / V ) in that case [33] is expected to be about an order of magnitude smaller (no pressure was applied on the spherical particle), and the beam current density ( J =7.3 ∼ 17.6 A cm −2 ) is more than two orders of magnitude higher than our case. According to equation (1), it is not surprising that an ∼ 100 K temperature increase was observed in their sample [33] . However, even such a temperature rise would be inconsequential in our case, because the T g for silica is rather high at ∼ 1,373 K and flow is not expected to be obvious at temperatures well below ∼ 0.7 T g . For our tensile test of NW, the sample was tangled and fixed at the crack of a colloidal film coated with carbon (graphite), an excellent thermal conductor. The NW between the two fixing ends has dimensions of 40 nm (diameter)× ∼ 5 μm (length), and the beam current density is 1.5×10 −4 to 1×10 −2 A cm −2 during tensile pulling. For the temperature difference Δ T to reach 100 K at the interface of the NW and the colloidal thin film (CTF), the actual contact area A should be smaller than 4 nm 2 (equation 1). However, the real contact area is expected to be much larger (that is, resulting in Δ T much lower than 100 K), because the NW is under large tensile stress that pulls the NW against the film substrate. The temperature difference inside the NW due to the equilibrium temperature gradient can be estimated using equation (2). Using the sample length of 5 μm, the maximum temperature difference along the NW is on the order of 0.1 K. Note that the above estimation assumed thermal equilibrium for the heat flow out of the sample, and used the thermal conductivity of bulk silica glass. These may not be completely correct assumptions for our experiments. For example, the thermal conductivity of a nanosized material may be lower than its bulk value; reduction up to two orders of magnitude was observed in crystalline silicon NWs because of surface phonon scattering [34] . However, in silica glass, wherein the mean free path of phonons is severely shortened by the amorphous structure, as shown by its low thermal conductivity, the additional impact of surface scattering and the size-induced reduction could be small. Even if the negligible temperature rise derived from the model may have underestimated the real temperature in the samples, it still can be concluded that the superplastic deformation in our experiments was observed at a temperature not significantly higher than RT, and clearly well below 0.7 T g . Next, we discuss the e-beam effects in promoting the dramatic plastic flow observed. We start from the mechanism mediating plastic deformation in silica. To acquire insight into how amorphous silica deforms under high stresses at RT, molecular dynamic (MD) simulations were performed (see Methods for details) for a very thin NW (diameter ∼ 3.6 nm). Large ductility was observed, which is not surprising because a significant fraction of atoms reside close to the surface, a natural imperfection with defects, vacancies and dangling bonds. We observe that the broken/dangling bonds reform with other neighboring atoms, accompanied by the rotation and migration of the atomic clusters involved. The repetition and accumulation of such bond-switching events cause plastic flow in the NW, healing incipient voids before their coalescence and giving rise to the observed ductility. A close-up view highlighting the Si-O bonds in action is given in Fig. 6a–c . We see that the broken bond creates a dangling silicon bond and a non-bridging oxygen atom. The non-bridging oxygen bonds with a different silicon, and at the same time the latter silicon severs bonding with another oxygen. The SiO 4 unit clusters are rotated and relocated as a result. Note that the same bond-switching mechanism has been proposed to explain the flow in viscous silica at high temperatures [5] and the voids coalescence under hydrostatic tension [12] . 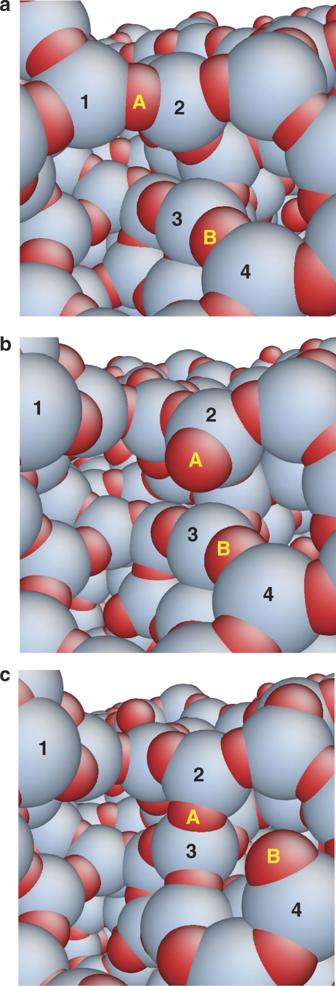Figure 6: A representative bond-switching event revealed by molecular dynamic (MD) simulations. 1–4 are silicon atoms, and A and B are oxygen atoms. The Si-O bonding (1–A) in panelais broken to create a silicon dangling bond 1-, and a non-bridging oxygen atom A- in panelb. Inc, the A- reforms bonding with 3, exposing B as a new non-bridging oxygen atom. The continuous occurrence and relay of such events lead to the creation and migration of dangling silicon bond and non-bridging oxygen atom, as well as the rotation and relocation of SiO4clusters. Figure 6: A representative bond-switching event revealed by molecular dynamic (MD) simulations. 1–4 are silicon atoms, and A and B are oxygen atoms. The Si-O bonding (1–A) in panel a is broken to create a silicon dangling bond 1-, and a non-bridging oxygen atom A- in panel b . In c , the A- reforms bonding with 3, exposing B as a new non-bridging oxygen atom. The continuous occurrence and relay of such events lead to the creation and migration of dangling silicon bond and non-bridging oxygen atom, as well as the rotation and relocation of SiO 4 clusters. Full size image In our experimental samples, which are much thicker, the vast majority of atoms are not close to surfaces. However, the mechanism revealed in the MD simulation above, that is, the atomic-scale 'repair' processes enabled by the prevalent bond switching, acquires help from electron radiation effects. During the e-beam irradiation, the first defect process in amorphous SiO 2 is the ionization damage due to electron–electron interaction, giving rise to Auger processes and bonding changes. This can lead to the cleavage of Si-O bond (its bond energy is in the range of 4.4–6.2 eV [19] , [35] ), forming a silicon and oxygen dangling bond pair. The second damage mechanism is the displacement of a bridging oxygen atom to form an interstitial oxygen atom, leaving behind a vacancy [36] . The displacement energy in amorphous silica is ∼ 25 eV [37] , reachable by the energy transferred from the 200 keV electron to oxygen (33 eV) and silicon (19 eV) [38] during an elastic collision. The radiation [7] , [36] , [39] , [40] thus leads to the formation of dangling bonds, the creation of oxygen vacancies (point-defect-like entities in amorphous solids [40] ) and possibly even the release of some oxygen molecules (although the change in the overall composition is not detectable; Fig. 4l ). All these are expected to facilitate the bond severing and re-forming ( Fig. 6 ) and the plastic flow during the high-stress-induced straining. The high-energy electrons and the defects they created directly facilitate the atoms to overcome the energy barrier for bond switching, reducing the flow stress and mediating the very large ductility, that is, the superplastic behavior observed. Ionization-induced diffusion [39] and viscous flow mediated by point-defect-like 'flow defects' in amorphous solids [40] have also been discussed before. In contrast, only brittle behavior is expected for a bulk piece of fused silica glass at RT. In this case, without the assistance of either the electron radiation, or high temperature, or large fraction of defects due to surfaces, the repair process cannot keep up with the void opening process. In general, the same bond-switching mechanism as shown in Figure 6 can lead to plasticity under various conditions. (1) At high temperature ≳ T g , the bond switching is activated by thermal energy to sustain viscous flow. (2) In a very thin NW, bond switching can be initiated by the defects and dangling bonds near the surface. (3) In the current work, we have e-beam penetrating the entire sample to promote the defects for flow at RT, leading to superplasticity in much larger samples. All the above three cases have similar results and underlying mechanism, but the causes are completely different: high temperature for (1), surface defects and large surface-to-volume ratio for (2) and e-beam defect creation and bond manipulation for (3). The latter is a low-temperature flow process in lieu of the high-temperature viscous flow. We conclude that the conventionally brittle amorphous silica, when manufactured into nanoscale objects, can be readily made ductile by low-intensity e-beam irradiation that does not noticeably change the temperature. This is because the energetic beam will generate structural and bonding defects throughout the entire sample body to facilitate the bond-switching events that impart flexibility to the atomic clusters, for their rotation and migration to accommodate the flow. In addition, when the sample is very small, it will be sufficiently flaw-free to sustain the high stresses (a few GPa) that are required to switch the bonds and relocate the clusters to annihilate any newly emerging damages. This atomic-level repair process heals the incipient voids that emerge on deformation, before they reach the critical size for crack initiation. 'Cold' superplastic deformation is thus made possible near RT, almost equivalent to flow near or above T g . In other words, the atomic-scale mechanism [5] , [12] , [13] responsible for the high-temperature thermally induced viscous flow is now rendered pronounced at RT with the help of the e-beam-induced defects. These results may open new avenues for the applications of brittle materials such as oxide glasses, and also have implications for their processing and integrity, as they are being scaled down into the nanometer regime in devices [1] , [2] . Although only silica glasses are studied here, we believe the e-beam effect on plastic deformation is general and may explain the large ductility previously observed inside TEM for other covalent or ionic brittle materials [41] . Our current discovery also expands the application of the e-beam in material processing and shaping, especially in bottom-up processes, because of the low beam density needed, the small temperature rise and the relatively large (at least submicron) samples that can be handled. TEM is used frequently for examining nanomaterials and for in situ testing of their properties. Our finding therefore provides the much-needed quantitative assessment of the e-beam effect on the plastic deformability of the material being illuminated, which has remained unexplored till now. Sample preparation Amorphous silica particles were produced by a sol–gel process. In a typical synthesis, 4 ml tetraethyl orthosilicate was injected into a mixture of 16 ml of distilled water, 4 ml of ammonium hydroxide and 80 ml isopropanol at RT under magnetic stirring. After reacting for 2 h, the colloidal spheres were collected by centrifugation, re-dispersed in 30 ml absolute ethyl alcohol. An additional thin layer of titania ( ∼ 10 nm) was deposited by using tetrabutyl titanate as the precursor and hydroxypropyl cellulose as the surfactant by following a procedure that we reported previously [42] . The products were washed with ethanol several times, and finally dried at 333 K for 8 h. The particles were ultrasonically dispersed in a dehydrated alcohol solution for 30 min. The solution containing the amorphous silica nanospheres was deposited on a silicon wedge substrate by a glass nebulizer, and some of the solid particles were left behind on top of the wedge plateau ( ∼ 1.5 μm in width) after the solvent evaporated. These particles are ∼ 500 nm in diameter. The type of silica glass studied in tensile testing was the amorphous silica fabricated using the popular thermal evaporation fabrication method [43] , [44] . Commercial high-purity (99.99 at%) silicon mono-oxide powder was used as the evaporation source. A silicon wafer was used as the substrate to collect the NWs. Together with the evaporation source, the silicon substrate was placed into the Al 2 O 3 container in a furnace at an inclined angle. No carbon source or other possible contaminations were involved in the synthesizing process of the NWs. The container was evacuated to a pressure of about 10 Pa, and back filled with Argon to ∼ 0.27×10 5 Pa. When conducting the thermal evaporation process, the heating rate was controlled to be a constant until the temperature reached 1,223 K. The system was kept at 1,223 K for 15 min and then cooled down to RT. A large amount of white cotton-like NWs were then collected from the silicon substrate. Microscopy and in situ testing JEOL FEG scanning electron microscope (JEOL 6500 SEM) and a JEOL FEG high-resolution TEM (HRTEM) operating at 200 keV were used to characterize the synthesized materials. The point resolution of the high-resolution TEM is about 0.19 nm. The electron energy dispersive spectrum and the EELS were taken with the JEOL 2010 FEG HREM, using a Gatan EELS attachment (Gatan). The energy resolution of the EELS system is about 1.2 eV. The fabricated silica NWs were found from these techniques to have properties similar to those reported by others [45] , [46] , [47] , [48] , [49] . From HREM images, we did not see any small-scale porosity that could cause measurable density changes in the NWs. The NWs were fabricated at high temperatures above 1,273 K, and no H 2 O molecules are expected inside the sample. From both of energy dispersive spectrum and EELS analysis, no obvious impurities were noticed, including chlorine. For compression testing on individual particles, the experiments were carried out in situ inside the TEM using the Hysitron PicoIndenter [16] , [17] . This quantitative technique is able to compress individual particle between a flat diamond punch and a flat silicon substrate, acquiring force-displacement data with ∼ 0.3 μN and ∼ 1 nm resolution, while simultaneously observing the deformation behavior in a TEM. The deformation process, in the displacement-controlled mode with a rate 10 nm s −1 , is recorded at 30 frames per s. See Supplementary Movie 1 . A multiple loading–partial unloading procedure was used for the mechanical testing, which improves the contact between the diamond punch and the particles for reproducible data and thermal conductance. For tensile testing, the NWs, with diameters about 40 nm, were on a specimen-supporting grid covered with CTF. 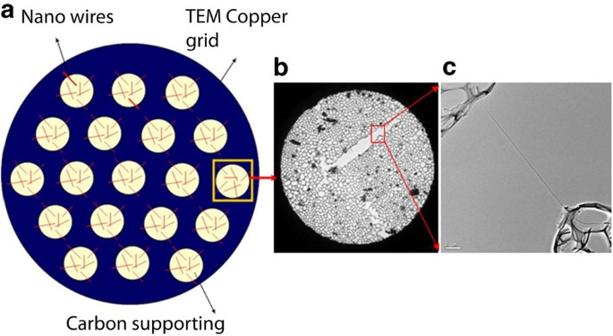Figure 7: The colloidal thin film contraction method for generating a tension force on the nanowires (NWs)21,22. (a) A sketch of the transmission electron microscope (TEM) copper grid. (b) One hole of the TEM grid with carbon-supporting film. (c) Pulling of a single NW by contracting the carbon film holding the NW. Figure 7 shows the details of this method [21] , [22] . Fig. 7a is an illustration of the TEM copper grid with a diameter of 3 mm. Fig. 7b shows one hole of the TEM grid, which was covered with a thin colloidal film for supporting the NW specimen. Cracks were made on the CTF, as shown in Figure 7b . The SiO 2 NWs spread-on were randomly scattered over the CTF, bridging the cracks. The two ends, A and B of one NW, were tangled and fixed in the cracked CTF, as shown in Figure 7c taken from the red-boxed region. With the e-beam illumination, the CTF shrank, applying axial-tensile stress on the SiO 2 NW. During the tensile pulling process, the e-beam was often moved away from the NWs. This is because the colloidal films require continued illumination to shrink further. The beam current density used for tensile pulling (illuminating the CTF) was usually from 1.5×10 −4 to 1×10 −2 A cm −2 . A flux of 4 A cm −2 was used for capturing the high-magnification HREM images (such as the case at a magnification of 400 000×). Figure 7: The colloidal thin film contraction method for generating a tension force on the nanowires (NWs) [21] , [22] . ( a ) A sketch of the transmission electron microscope (TEM) copper grid. ( b ) One hole of the TEM grid with carbon-supporting film. ( c ) Pulling of a single NW by contracting the carbon film holding the NW. Full size image MD simulations Molecular dynamics simulations using large-scale atomic/molecular massively parallel simulator (LAMMPS) [50] were performed using the Carre–Horbach–Ispas–Kob (CHIK) potential [51] , which is a modified version of the classical Beest–Kramer–Santen (BKS) potential [52] . The simulation box contains 6,000 atoms (2,000 silicon and 4,000 oxygen), with dimensions of 3.56 nm ( x ) ×3.56 nm ( y ) ×7.12 nm ( z ) (density 2.2 g cm −3 ). The samples were intially melted and equilibrated at 6,000 K for 100 ps, and then quenched to 300 K under the NVT (constant number of particles, volume and temperature) condition at 5 K ps −1 . The temperature was scaled with cooling and controlled by Nose–Hoover thermostat, as implemented in LAMMPS. Uniaxial tensile tests were conducted, with periodic boundary condition applied along the z (length) direction, and relaxed free surfaces for the x and y directions. Temperature for the loading tests was controlled at 300 K. Deformation was applied by scaling the simulation box at a step size of ∼ 0.001% tensile strain, followed by structural relaxation at 300 K. The uniaxial strain rate along the z direction is ∼ 10 8 s −1 . How to cite this article: Zheng K. et al . Electron-beam-assisted superplastic shaping of nanoscale amorphous silica. Nat. Commun. 1:24 doi: 10.1038/1021 (2010).